A general method for the large-scale synthesis of uniform ultrathin metal sulphide nanocrystals Ultrathin metal sulphide nanomaterials exhibit many unique properties, and are thus attractive materials for numerous applications. However, the high-yield, large-scale synthesis of well-defined ultrathin metal sulphide nanostructures by a general and facile wet-chemical method is yet to be realized. Here we report a universal soft colloidal templating strategy for the synthesis of high-quality ultrathin metal sulphide nanocrystals, that is 3.2 nm-thick hexagonal CuS nanosheets, 1.8 nm-diameter hexagonal ZnS nanowires, 1.2 nm-diameter orthorhombic Bi 2 S 3 nanowires and 1.8 nm-diameter orthorhombic Sb 2 S 3 nanowires. As a proof of concept, the ultrathin CuS nanosheets are used to fabricate an electrode for a lithium-ion battery, which exhibits a large capacity and good cycling stability, even after 360 cycles. Furthermore, high-yield, gram-scale production of these ultrathin metal sulphide nanomaterials has been achieved (~100%, without size-sorting process). Our method could be broadly applicable for the high-yield production of novel ultrathin nanostructures with great promise for various applications. The rise of graphene [1] , [2] has recently inspired great research interest in other types of ultrathin nanomaterials [3] , [4] , [5] . Ultrathin nanostructures are considered to have at least one dimension approaching the size of one or two crystal unit cells, typically in the sub-5 nm regime [6] , [7] , [8] , [9] . Increasing interest in ultrathin nanomaterials is due to their attractive properties and various potential applications [6] , [7] , [8] , [9] . In particular, ultrathin metal sulphide nanocrystals have drawn tremendous attention owing to their unique properties arising from their exceptionally small dimensions and the resultant quantum size effects [10] , [11] , [12] , [13] , [14] , [15] , [16] . Importantly, the easy preparation and processability of these nanostructures makes them promising building blocks for a wide range of applications. To effectively synthesize such ultrathin nanostructures via colloidal chemical synthesis, the delicate manipulation of the interaction between crystal nuclei and ligand molecules is necessary as this may realize the anisotropic growth of the nanocrystals along one specific orientation. Up to now, several ultrathin metal sulphide nanostructures have been prepared via organometallic or organic solution phase synthesis. Examples include the sub-2 nm-diameter Cu 2 S (ref. 10 ), ZnS (refs 11 , 12 ), Bi 2 S 3 (ref. 13 ) and Sb 2 S 3 (ref. 14 ) nanowires, and sub-2 nm-thick hexagonal β−In 2 S 3 nanoplates [15] and ZrS 2 nanodiscs [16] . However, a general and facile method for the large-scale synthesis of well-defined ultrathin metal sulphide nanostructures has not been demonstrated, which inspires the continuous and systematic exploration. Here we report a simple and general approach towards the large-scale synthesis of ultrathin metal sulphide nanocrystals based on the soft-templating strategy. For example, the monodisperse, ultrathin, single-crystal CuS nanosheets, with a thickness of ~3.2 nm (two unit cells) and plane size up to ~453 nm (aspect ratio up to 150), have been synthesized in large amounts. Moreover, our general method has been successfully used for the synthesis of other ultrathin metal sulphide nanocrystals, such as sub-2 nm-diameter hexagonal ZnS, orthorhombic Bi 2 S 3 and orthorhombic Sb 2 S 3 nanowires. Synthesis and characterization of ultrathin CuS nanosheets To synthesize ultrathin CuS nanostructures, 1.5 mmol of copper (I) chloride (CuCl) was added to a mixture of 5 ml oleylamine (OM) and 5 ml octylamine (OTA) in a three-necked flask (100 ml) at room temperature. The slurry was heated to 100 °C with vigorous magnetic stirring under vacuum for ~30 min in a temperature-controlled electromantle to remove water and oxygen. The temperature was maintained at 130 °C for 4 h and the solution became transparent. Then, the sulphur (S) dispersion formed by ultra-sonication of 4.5 mmol of S powder in the mixture of 2.5 ml OTA and 2.5 ml OM at room temperature was quickly injected into the resulting solution at 95 °C. The resulting mixture was kept at 95 °C for 18 h, and it became dark. After it cooled to room temperature, the CuS nanosheets were precipitated by adding the excess absolute ethanol (~40 ml) into the solution. The synthesized CuS nanostructures possess a hexagonal phase (covellite type, space group P63/mmc), as confirmed by the powder X-ray diffraction analysis ( Supplementary Fig. S1a ), with the calculated lattice constants of a = b =3.76 Å and c =16.21 Å (JCPDS 78−0877). The Raman spectrum of the CuS nanostructures shows a distinct band at 474 cm −1 ( Supplementary Fig. S1b ), which originates from the lattice S−S stretching of covellite [17] . The morphology of the as-obtained CuS nanostructures was observed by field emission scanning electron microscopy ( Fig. 1a–c ) and transmission electron microscopy (TEM, Fig. 1d ). The field emission scanning electron microscopy image in Fig. 1a demonstrates the formation of uniform CuS nanosheets with a very high purity (yield of ~100%). Some nanosheets self-assembled into the domino-like superstructures through face-to-face stacking along the c axis ( Fig. 1b ). The stacked CuS nanosheets can be disassembled to individual ones upon transferring to an aqueous solution via a simple surface modification and extraction process (see the Methods section for details). 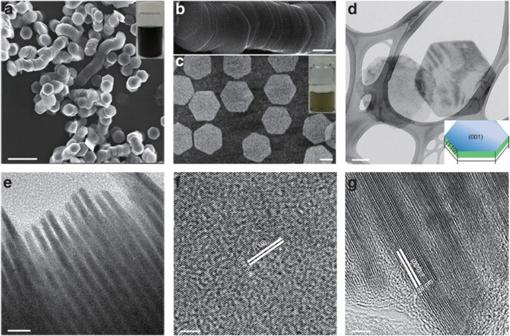Figure 1: Field emission scanning electron microscopy (FESEM) and TEM images of ultrathin CuS nanosheets. FESEM images of (a) ultrathin CuS nanosheets (inset: photograph of the as-prepared colloid solution of CuS nanosheets, scale bar=1 μm), (b) domino-like superstructures of the ultrathin CuS nanosheets (scale bar=200 nm) and (c) free-standing uniform ultrathin monolayer CuS nanosheets on Si substrate (inset: photograph of individual CuS nanosheets dispersed in Milli-Q water, which has been kept in ambient conditions for >3 months, scale bar=200 nm). TEM images of ultrathin CuS nanosheets with (d) lying flat (scale bar=100 nm) and (e) standing (scale bar=10 nm) on the TEM grids. Inset ind: a scheme for an ultrathin CuS nanosheet. High-resolution TEM images of (f) an individual CuS nanosheets (scale bar=1 nm) lying flat and (g) several stacked ultrathin CuS nanosheets (scale bar=2 nm) standing on the TEM grids. Figure 1c clearly reveals the free-standing, individual ultrathin CuS nanosheets. The obtained aqueous solution is stable in ambient conditions for >3 months (inset in Fig. 1c ). Figure 1d show the TEM images of hexagonal CuS nanosheets lying flat and standing perpendicularly on copper grids, respectively. The high-resolution TEM images ( Fig. 1f ) prove that the nanosheets are single-crystalline. The observed interplane distances between the lattice fringes are ~0.18 and ~0.26 nm, corresponding to the (110) and (006) planes of CuS, respectively. Thus, the obtained CuS nanosheets preferably grow normal to the <001> direction, and exhibit an exceptionally high aspect ratio with average plane length of 453±6 nm and thickness of 3.2±0.2 nm, corresponding to two unit cells (the lattice constant of the unit cell of CuS is about 1.6 nm, Supplementary Fig. S2 ). Interestingly, TEM images also show the Moiré patterns caused by the interference between the crystalline lattices of the stacked nanosheets ( Supplementary Fig. S3 ). As observed from a typical CuS nanosheet array aligned along the <001> direction in Fig. 1e , the distance between the adjacent nanosheets is ~2 nm, implying the retention of capping ligands on the nanosheets surfaces, which was also confirmed by the Fourier transform infrared and X-ray photoelectron spectroscopy (XPS) spectra in Supplementary Fig. S4 . Note that some nanosheets are bent on the TEM grid ( Supplementary Fig. S5 ), indicating the highly flexible nature of the ultrathin CuS nanosheets. The XPS ( Supplementary Fig. S6 ) and energy-dispersive X-ray spectroscopy ( Supplementary Fig. S7 ) data confirmed the formation of the stoichiometric CuS compound. Figure 1: Field emission scanning electron microscopy (FESEM) and TEM images of ultrathin CuS nanosheets. FESEM images of ( a ) ultrathin CuS nanosheets (inset: photograph of the as-prepared colloid solution of CuS nanosheets, scale bar=1 μm), ( b ) domino-like superstructures of the ultrathin CuS nanosheets (scale bar=200 nm) and ( c ) free-standing uniform ultrathin monolayer CuS nanosheets on Si substrate (inset: photograph of individual CuS nanosheets dispersed in Milli-Q water, which has been kept in ambient conditions for >3 months, scale bar=200 nm). TEM images of ultrathin CuS nanosheets with ( d ) lying flat (scale bar=100 nm) and ( e ) standing (scale bar=10 nm) on the TEM grids. Inset in d : a scheme for an ultrathin CuS nanosheet. High-resolution TEM images of ( f ) an individual CuS nanosheets (scale bar=1 nm) lying flat and ( g ) several stacked ultrathin CuS nanosheets (scale bar=2 nm) standing on the TEM grids. Full size image Optical properties of ultrathin CuS nanosheets The optical properties of the synthesized ultrathin CuS nanosheets are characterized by ultraviolet (UV)–vis-near infrared (NIR) absorption and photoluminescence (PL) spectroscopy. 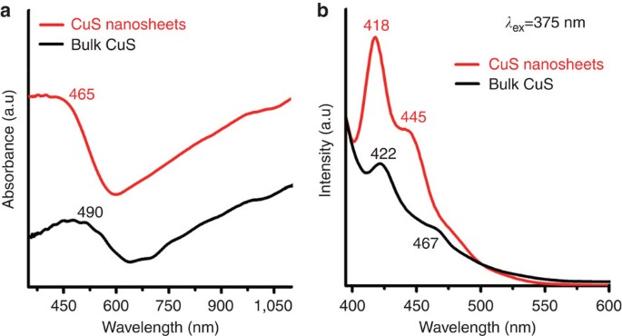Figure 2: Optical properties of ultrathin CuS nanosheets. (a) UV–vis-NIR absorption spectra of as-obtained ultrathin CuS nanosheets and its bulk counterpart. (b) Room temperature PL spectra of ultrathin CuS nanosheets and its bulk counterpart underλex=375 nm. Figure 2a depicts the UV–vis-NIR spectra of the ultrathin CuS nanosheets and its bulk counterpart (obtained directly from the vigorous sonication of commercial CuS in ethanol for about 30 min, Supplementary Fig. S8 ). Both of their spectra show a strong absorption in the near infrared region, characteristic of covellite [18] . A discernible absorption peak is detected in the visible region at 465 nm, which is the lowest energy excitonic absorption peak of CuS nanosheet. The lowest energy exciton transition peak of CuS nanosheets exhibits a blue shift when compared with the absorption peak of bulk CuS (490 nm). Figure 2b shows the emission spectra of the ultrathin CuS nanosheets and their bulk counterpart under λ ex =375 nm. Relative to the PL spectra of the bulk (emission at 422 and 467 nm), the stronger and narrower emission peaks at 418 and 445 nm of the ultrathin CuS nanosheets also present a clear blue shift. The sharp absorption and emission peaks, along with the distinct blue shift, imply that our synthesized CuS nanosheets not only are uniform in size and morphology, but also exhibit the strong quantum confinement effects due to their ultra-small thickness. Figure 2: Optical properties of ultrathin CuS nanosheets. ( a ) UV–vis-NIR absorption spectra of as-obtained ultrathin CuS nanosheets and its bulk counterpart. ( b ) Room temperature PL spectra of ultrathin CuS nanosheets and its bulk counterpart under λ ex =375 nm. Full size image Li-ion battery performance of ultrathin CuS nanosheets As a well-known p-type semiconductor, CuS is one of the most intensively studied materials because of its diverse applications in the fields of Li-ion batteries, solar cells, nonlinear optical materials and so on [19] , [20] , [21] , [22] . The layered structure of CuS is composed of copper atoms sandwiched between two layers of hexagonally close-packed S atoms. This crystallographic feature allows for the intercalation and reaction of alkali metal ions in between the S–Cu–S layers, making the CuS nanosheet a promising electrode material for Li-ion battery applications. 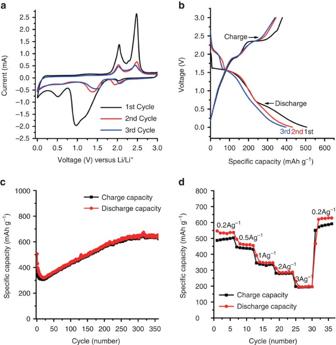Figure 3: Li-ion battery performance of ultrathin CuS nanosheets. (a) CV curves of CuS electrode at a scanning rate of 0.5 mV s−1over a voltage range of 0.005−3.0 V. (b) Charge–discharge voltage profiles of the CuS nanosheets electrode at a current density of 0.2 A g−1for the first three cycles. (c) Cycling performance of the CuS electrode tested at a current density of 0.2 A g−1within a voltage window of 0.005−3.0 V. (d) Cycling performance of the CuS nanosheets electrode at various current density. Figure 3a depicts the representative cyclic voltammograms (CVs) of a CuS electrode at a scan rate of 0.5 mV s −1 for the first, second and third cycles, which demonstrates the redox reactions during the charge–discharge process. Two pairs of distinct redox current peaks can be clearly identified from the CV curves, for example oxidation peaks at around 2.0 and 2.5 V. The typical charge–discharge cycling performance of the Li-ion battery based on the synthesized CuS was evaluated between 0.005 and 3.0 V at a current density of 0.2 A g −1 . Figure 3b shows the charge–discharge voltage profiles of the CuS electrode for the first three cycles at a current rate of 0.2 A g −1 . The first intercalation process gives a discharge capacity of 506 mAh g −1 and a corresponding charge capacity of 378 mAh g −1 . During the second cycle, the electrode displays a discharge capacity of 431 mAh g −1 , where the charge capacity is 344 mAh g −1 . The electrode presents a discharge capacity of 396 mAh g −1 in the third discharge process, where the charge capacity is 339 mAh g −1 . In Fig. 3c , it is observed that the discharge capacity decreased from 506 mAh g −1 at the first cycle to 321 mAh g −1 at the 20th cycle and then increased to a higher value of 642 mAh g −1 at the 270th cycle. The capacity is sustained to the 360th cycle, which suggests the good cyclability of the CuS electrode compared with those reported previously [23] , [24] , [25] . The increase of capacity from the 20th to the 270th cycle indicates a possible activation process in the electrode material. Accordingly, this increase in capacity was accompanied by the decrease of the electrode impedance as shown in the Supplementary Fig. S9 . The CuS nanosheet electrode was also evaluated at high current densities, which delivers capacities as high as 285 and 198 mAh g −1 at the current densities of 2 and 3 A g −1 , respectively ( Fig. 3d ). Moreover, we also examined the structure of the electrode material during the repeated cycles to explain the observed cycling performance of the CuS electrode ( Supplementary Fig. S10 ). Figure 3: Li-ion battery performance of ultrathin CuS nanosheets. ( a ) CV curves of CuS electrode at a scanning rate of 0.5 mV s −1 over a voltage range of 0.005−3.0 V. ( b ) Charge–discharge voltage profiles of the CuS nanosheets electrode at a current density of 0.2 A g −1 for the first three cycles. ( c ) Cycling performance of the CuS electrode tested at a current density of 0.2 A g −1 within a voltage window of 0.005−3.0 V. ( d ) Cycling performance of the CuS nanosheets electrode at various current density. Full size image To study the formation mechanism of the ultrathin CuS nanosheets, we propose that the CuCl(OTA, OM) x lamellar structure ( x : the total number of N atoms in OTA and OM molecules coordinated with Cu atom in the reaction) is first formed by the reaction of CuCl, OTA and OM. The as-observed growth of the ultrathin CuS nanosheets is attributed to the templating effect of the formed micellar structures ( Fig. 4 ) [8] . Such a template-guided growth mechanism is confirmed by the following control experiments. After addition of acetone to the mixture of CuCl, OTA and OM, followed by centrifugation, the precipitate was collected. The 1 H NMR ( Supplementary Fig. S11 ) confirms the presence of OM ligands in the CuCl(OTA, OM) x intermediate. The TEM image of the CuCl(OTA, OM) x solid collected upon precipitation shows the formation of arrayed strands ( Supplementary Fig. S12a ). The weak contrast of the strands in the TEM image indicates that they are mainly composed of organic species ( Supplementary Fig. S12a ). Supplementary Figure S12b shows the small-angle X-ray diffraction (SAXRD) pattern of the obtained precipitate, confirming that the complex has a typically lamellar structure. A series of SAXRD peaks could be assigned to ‘00L’ ( L =1, 2, 3, 4...) with a layer spacing of ~3.8 nm, which is consistent with the combined length of OTA (the molecule length of 1.35 nm) and OM (the molecule length of 2.5 nm). Note that the lengths of OTA and OM molecules were calculated according to the formula, L (nm)=0.25+0.127 n [26] , where n is the number of carbon atoms in the alkyl chain. The micellar-templating mechanism proposed in our work was also used to explain the formation of ultrathin FePt nanowires [27] , barium sulphate nanofilaments [28] and Au nanowires [8] , [29] , [30] . 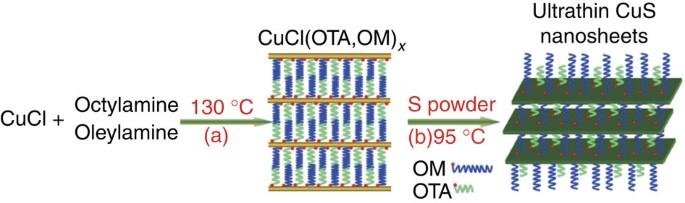Figure 4: Schematic illustration of synthesis of ultrathin CuS nanosheets. Step (a): The (CuCl(OTA, OM)x) lamellar complex is formed by the reaction of CuCl, OTA and OM at 130 °C. Step (b): (CuCl(OTA, OM)x) lamellar complex acts as the soft template for synthesis of ultrathin CuS nanosheets after addition of S powder. Figure 4: Schematic illustration of synthesis of ultrathin CuS nanosheets. Step (a): The (CuCl(OTA, OM) x ) lamellar complex is formed by the reaction of CuCl, OTA and OM at 130 °C. Step (b): (CuCl(OTA, OM) x ) lamellar complex acts as the soft template for synthesis of ultrathin CuS nanosheets after addition of S powder. Full size image Note that we have conducted a series of experiments to optimize the conditions for synthesis of high-quality ultrathin CuS nanosheets. In our experiment, we found that the concentration of precursors, the composition of solvents, and the reaction temperature and time play important roles in the formation of uniform CuS nanosheets. For example, if the volume of solvents and the concentration (4.5 mmol) of S precursor were fixed, when high concentration (4.5 mmol) or low concentration (0.5 mmol) of CuCl was used for the reaction at 95 °C for 18 h, the non-uniform CuS nanosheets were obtained ( Supplementary Fig. S13 ). Besides the precursor concentration, we found that the equal volume mixture of OTA and OM is essential for the preparation of uniform CuS nanosheets. For example, if either OTA/OM=3/1 (v/v) or OTA/OM=1/3 (v/v) was used as the mixed solvent, aggregated CuS nanosheets formed together with a great amount of nanoparticles ( Supplementary Fig. S14 ). In addition, we also found that both the reaction temperature and time remarkably affect the quality of the products. For example, at fixed experimental conditions, that is 1.5 mmol CuCl, OTA/OM=1/1 (v/v) and a reaction time of 18 h, when the reaction temperature decreased from 95 to 50 °C, almost no solid matter appeared after the precipitation treatment ( Supplementary Fig. S15a ), indicating the deficient energy for the formation of CuS nanosheets. However, as the temperature increased to 160 °C, the non-uniform CuS nanoparticles were obtained ( Supplementary Fig. S15b ). On the other hand, at the fixed reaction temperature (95 °C), the reaction of 1.5 mmol CuCl in OTA/OM (1:1, v/v) for a short reaction time (for example, t =3 h) resulted in irregular CuS nanoparticles ( Supplementary Fig. S16a ). At t =6 h, only some unshapely flake-like nanostructures were obtained ( Supplementary Fig. S16b ). When the reaction time was in the range of 9–12 h, the nanosheets were discernible but the shape was not uniform ( Supplementary Fig. S16c ,d). After 12 h, the size and size distribution of as-obtained uniform CuS nanosheets did not change significantly ( Supplementary Fig. S16e ), suggesting a drastic ‘size-defocusing’ process [31] . However, when the reaction ran for 24 h, aggregated CuS nanosheets were observed ( Supplementary Fig. S16f ), indicating a distinct ‘Ostwald ripening’ process [32] , [33] . Importantly, our synthetic approach based on the soft-templating effect is widely applicable. We have successfully used it to synthesize a series of ultrathin metal sulphide nanostructures. For example, when zinc chloride (ZnCl 2 ) was refluxed in a solution containing OTA and dodecylamine (DDA) ( Supplementary Fig. S17 ), the uniform ZnS nanowires with an average diameter of 1.8 nm were synthesized, exhibiting a blue PL under UV excitation ( Fig. 5a–c ). Similarly, when precursors such as bismuth (III) chloride (BiCl 3 ) or antimony (III) chloride (SbCl 3 ) were refluxed in solutions containing OTA and OM ( Supplementary Figs S18 and S19 ), the uniform 1.2 nm-diameter Bi 2 S 3 nanowires ( Fig. 5d ) or 1.8 nm-diameter Sb 2 S 3 nanowires ( Fig. 5e ) were also synthesized. The nanowires were further confirmed by a set of tilted TEM images ( Supplementary Figs S20, S21 and S22 ). Most importantly, our synthetic procedure for preparation of ultrathin metal sulphide nanostructures can be readily reproduced and scaled up. For example, to demonstrate the large-scale synthesis, we performed the reaction with 30 mmol of CuCl precursor and obtained as much as ~1.4 g of ultrathin CuS nanosheets in a single batch without a size-sorting process ( Supplementary Fig. S23 ). In addition, ~1.3 g ultrathin ZnS nanowires with hexagonal phase ( Supplementary Fig. S24 ), ~1.6 g ultrathin Bi 2 S 3 nanowires with orthorhombic phase ( Supplementary Fig. S25 ) and ~1.7 g ultrathin Sb 2 S 3 nanowires with orthorhombic phase ( Supplementary Fig. S26 ) have been successfully synthesized via the one-pot process. 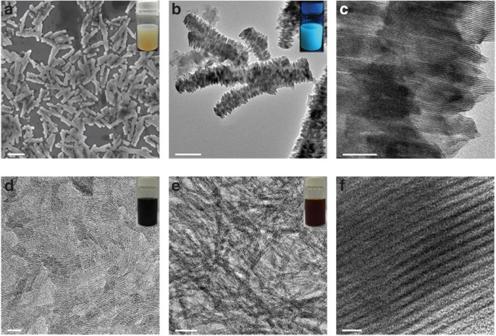Figure 5: Field emission scanning electron microscopy (FESEM) and TEM images of ultrathin metal sulphide nanostructures. (a) FESEM images of ultrathin ZnS nanowire assemblies (scale bar=2 μm). Inset: photograph of ultrathin ZnS nanowire solution. (b) TEM image of ultrathin ZnS nanowires (scale bar=500 nm). Inset: photograph of ultrathin ZnS nanowire solution excited with a UV lamp at 365 nm. (c) TEM image of ultrathin ZnS nanowires with diameter of 1.8 nm (scale bar=50 nm). (d) TEM images of ultrathin Bi2S3nanowires with diameter of 1.2 nm (scale bar=20 nm). Inset: photograph of ultrathin Bi2S3nanowire solution. (e) TEM image of ultrathin Sb2S3nanowires (scale bar=100 nm). Inset: photograph of ultrathin Sb2S3nanowire solution. (f) TEM image of ultrathin Sb2S3nanowires with diameter of 1.8 nm (scale bar=5 nm). Figure 5: Field emission scanning electron microscopy (FESEM) and TEM images of ultrathin metal sulphide nanostructures. ( a ) FESEM images of ultrathin ZnS nanowire assemblies (scale bar=2 μm). Inset: photograph of ultrathin ZnS nanowire solution. ( b ) TEM image of ultrathin ZnS nanowires (scale bar=500 nm). Inset: photograph of ultrathin ZnS nanowire solution excited with a UV lamp at 365 nm. ( c ) TEM image of ultrathin ZnS nanowires with diameter of 1.8 nm (scale bar=50 nm). ( d ) TEM images of ultrathin Bi 2 S 3 nanowires with diameter of 1.2 nm (scale bar=20 nm). Inset: photograph of ultrathin Bi 2 S 3 nanowire solution. ( e ) TEM image of ultrathin Sb 2 S 3 nanowires (scale bar=100 nm). Inset: photograph of ultrathin Sb 2 S 3 nanowire solution. ( f ) TEM image of ultrathin Sb 2 S 3 nanowires with diameter of 1.8 nm (scale bar=5 nm). Full size image In summary, we have successfully developed a general method for the large-scale, one-pot synthesis of uniform, ultrathin metal sulphide nanocrystals. This method, based on the soft-templating strategy, offers several advantages over conventional methods for the synthesis of ultrathin metal sulphide nanocrystals. First, it is a general process that can be used to synthesize different kinds of high-quality ultrathin metal sulphide nanocrystals with various compositions and phases, that is the 3.2 nm-thick hexagonal CuS nanosheets, 1.8 nm-diameter hexagonal ZnS nanowires, 1.2 nm-diameter orthorhombic Bi 2 S 3 nanowires and 1.8 nm-diameter orthorhombic Sb 2 S 3 nanowires. Second, in comparison with the organometallic thermo-decomposition and chemical vapour deposition methods for preparation of ultrathin metal sulphide nanocrystals, it is environmentally friendly and economical, as it uses the non-toxic, green phosphine-free and inexpensive reagents such as metal chlorides. Last, but by no means least, it enables the large-scale (grams), high-yield (~100%, without further size-sorting) synthesis of uniform ultrathin metal sulphide nanocrystals in a one-step process at a relatively low cost. We believe that our strategy could be broadly applicable for the facile and high-yield production of other novel ultrathin nanostructures with great promise for various applications. Chemicals Copper (I) chloride (CuCl, 99.995%, Sigma-Aldrich), zinc chloride (ZnCl 2 , >98%, Fluka), bismuth (III) chloride (BiCl 3 , >98%, Alfa Aesar), antimony (III) chloride (SbCl 3 , >99%, Sigma-Aldrich), sulphur powder (S, Sigma-Aldrich), oleylamine (OM, >80%, Sigma-Aldrich), octylamine (OTA, 99%, Sigma-Aldrich), 1-dodecylamine (DDA, >98%, Alfa Aesar), cetyltrimethylammonium bromide (CTAB, Sigma-Aldrich), ethanol (AR) and cyclohexane (AR) were used as received without further purification. Synthesis of ultrathin CuS nanosheets A typical procedure is described as follows: after 1.5 mmol of CuCl was added to the mixture of 5 ml OM and 5 ml OTA in a three-necked flask (100 ml) at room temperature, the slurry was heated to 100 °C to remove water and oxygen with vigorous magnetic stirring under vacuum for ~30 min in a temperature-controlled electromantle. After the solution was maintained at 130 °C for 4 h, it became transparent. Then, the S dispersion formed by ultra-sonication of 4.5 mmol of S powder in the mixture of 2.5 ml OTA and 2.5 ml OM at room temperature was quickly injected into the resulting solution at 95 °C. After the resulting mixture was kept at 95 °C for 18 h, it became dark. After it cooled down to room temperature, the CuS nanosheets were precipitated by adding excess absolute ethanol (~40 ml) to the solution. The CuS nanosheets were collected by centrifugation at 8,500 r.p.m. for 20 min. The as-formed CuS nanosheets were easily re-dispersed in various apolar organic solvents (for example cyclohexane, toluene). The yields of the obtained nanosheets were ca. 75–85%. Transfer hydrophobic CuS nanosheets to aqueous solution The hydrophobic CuS nanosheets could be further functionalized by various cationic surfactants such as CTAB through the ligand wrapped reaction, enabling the phase transfer of CuS nanosheets from hydrophobic to hydrophilic media. In a typical process, after 5 mg of hydrophobic CuS nanosheet powder was dispersed in 2 ml chloroform (~2.5 mg ml −1 ) to form a homogeneous colloidal dispersion, 2 ml of the aforementioned CuS colloid solution was added into 10 ml of CTAB solution (3.64 g ml −1 ). A subsequent ultra-sonication (~1 min) led to the stable white emulsion. After that, the stable emulsion was placed on a hotplate at 80 °C with a vigorous stirring for 15 min until a transparent solution was formed, indicating the successful binding of organic ligands to the nanosheets surface. After centrifugation to remove the free surfactants, the precipitated hydrophilic nanosheets were re-dispersed in Milli-Q water to form a stable dispersion. Synthesis of ultrathin ZnS nanowires The synthetic procedure was similar to that of CuS nanosheets, except that 1.5 mmol of ZnCl 2 and 4.5 mmol of S (dispersed in 2.5 ml of OTA and 2.5 ml of DDA), used as the precursors, were added into a mixture of OTA (5 ml) and DDA (5 ml) for a reaction at 100 °C for 18 h. Synthesis of ultrathin Bi 2 S 3 nanowires The synthetic procedure was similar to that of CuS nanosheets, except that 1.5 mmol of BiCl 3 and 4.5 mmol of S (dispersed in 2.5 ml of OTA and 2.5 ml of OM), used as the precursors, were added into a mixture of OTA (5 ml) and OM (5 ml) for a reaction at 140 °C for 18 h. Synthesis of ultrathin Sb 2 S 3 nanowires The synthetic procedure was similar to that of CuS nanosheets, except that 1.5 mmol of SbCl 3 and 4.5 mmol of S (dispersed in 2.5 ml of OTA and 2.5 ml of OM), used as the precursors, were added into a mixture of OTA (5 ml) and OM (5 ml) for a reaction at 150 °C for 18 h. Characterization Powder X-ray diffraction patterns of the dried powders were recorded on Bruker D8 diffractometer (German) with a slit of 1/2° at a scanning rate of 2° min −1 , using Cu K α radiation ( λ =1.5406 Å). The lattice parameters were calculated with the least-squares method. Samples for TEM analysis were prepared by drying a drop of nanocrystal dispersion in cyclohexane on amorphous carbon-coated copper grids. High-resolution TEM characterization was performed with a JEOL 2100F (Japan) operated at 200 kV. Room-temperature Raman spectra were measured with a WITec CRM200 confocal Raman microscopy system with the excitation line of 488 nm and an air cooling charge coupled device as the detector (WITec Instruments Corp, Germany). The Raman band of a silicon wafer at 520 cm −1 was used as the reference to calibrate the spectrometer. The small-angle X-ray diffraction (SAXRD) patterns were obtained on Rigaku D/MAX-2000 diffractometer (Japan) using Cu K α radiation ( λ =1.5418 Å). Small-angle X-ray scattering patterns of samples, contained in a 1 mm-diameter capillary holder, were collected using Anton Paar SAXess (40 kV, 50 mA, transmission geometry, Germany) with line focus at room temperature. The scanning time was 5 min for each sample. The patterns were collected with an imaging plate followed by scanning. Integration over 10 mm window was performed to transform the two-dimensional scattering patterns into one-dimensional data. The fluorescence spectra of the CuS nanosheets and the bulk powder were obtained on a Shimadzu/RF-5301PC fluorescence spectrometer (Japan) at room temperature. The UV–vis-NIR absorption spectra of the nanocrystals were obtained on a Shimadzu/UV-1800 UV–vis-NIR spectrometer (Japan). XPS was performed on a Kratos AXIS Ultra photoelectron spectrometer using Al KR radiation (1486.71 eV). The Fourier Transform Infrared absorption spectra of the nanocrystals were carried on Perkin Elmer/Spectrum GX FTIR Spectrometer (USA). The 1 H NMR characterization was recorded on Varian Mercury 200 MHz spectrometers (USA) with the number of transmittal of 64, and referenced to tetramethylsilane (TMS) as the internal standard. Electrochemical measurements The as-prepared CuS nanosheets were firstly annealed in Ar:H 2 (80%:20%, volume) for 5 min at 700 °C. Then, 80 wt% of the annealed CuS, 10 wt% P2-single-walled carbon nanotube and 10 wt% polyvinylidene fluoride binder were mixed using N -methyl-2-pyrrolidinone, and stirred for 12 h. The obtained slurry was then coated onto Cu foil disks and dried in vacuum at 50 °C for 12 h to remove the solvent to form the working electrode. Electrochemical measurement was carried out on the CR2032 (3 V) coin-type cells with Li metal as the counter/reference electrode, CELGARD 2400 membrane as the separator, and 1 M LiPF 6 in ethylene carbonate/diethyl carbonate (1:1 by the volume) was used as the electrolyte. The coin cells were assembled in an Ar-filled glove box with concentrations of moisture and oxygen below 1.0 p.p.m. The charge/discharge tests were performed in a NEWARE battery tester at a voltage window of 0.005−3.0 V for CuS samples. CV curves of CuS electrode was performed at a scanning rate of 0.5 mV s −1 in a voltage range of 0.005−3.0 V using an electrochemical workstation (CHI 660C). How to cite this article : Du Y. et al . A general method for the large-scale synthesis of uniform ultrathin metal sulfide nanocrystals. Nat. Commun . 3:1177 doi: 10.1038/ncomms2181 (2012).